Direct visualization of HIV-enhancing endogenous amyloid fibrils in human semen Naturally occurring fragments of the abundant semen proteins prostatic acid phosphatase (PAP) and semenogelins form amyloid fibrils in vitro. These fibrils boost HIV infection and may play a key role in the spread of the AIDS pandemic. However, the presence of amyloid fibrils in semen remained to be demonstrated. Here, we use state of the art confocal and electron microscopy techniques for direct imaging of amyloid fibrils in human ejaculates. We detect amyloid aggregates in all semen samples and find that they partially consist of PAP fragments, interact with HIV particles and increase viral infectivity. Our results establish semen as a body fluid that naturally contains amyloid fibrils that are exploited by HIV to promote its sexual transmission. Unprotected sexual intercourse is the main route for the dissemination of HIV in the human population, and semen is the most important vector for virus transmission [1] , [2] , [3] , [4] . To establish productive infection, HIV needs to access its target cells, mainly CD4+ T cells, macrophages or dendritic cells [1] , [2] , [3] , [4] . When analysed under conditions that minimize semen’s well-documented in vitro cytotoxicity [5] , [6] , [7] , [8] , [9] , semen markedly increases HIV attachment and infection of these cell types [10] , [11] , [12] , [13] , [14] , [15] , [16] , [17] . Thus, semen may not just be a passive carrier for HIV but also facilitate viral transmission [18] , [19] . The relative HIV-enhancing activity of individual semen samples strongly correlates with the levels of amyloidogenic peptides [13] , [17] . These peptides are derived from at least three abundant semen proteins, that is, prostatic acid phosphatase (PAP) [11] , [20] , and semenogelins (SEM) 1 and 2 (ref. 17) [17] . Freshly dissolved, chemically synthesized versions of these peptides have no effect on HIV infection. However, agitation of PAP248-286 (refs 11 , 12 , 13 , 14 , 15 , 16 , 21 ), PAP85-120 (ref. 20) [20] and SEM fragments [17] , results in the formation of amyloid fibrils, which potently increase viral infectivity. This phenomenon has previously also been observed in the case of Alzheimer’s disease-associated Aß fibrils 22 . The best-characterized seminal amyloid is PAP248-286, which forms fibrils termed SEVI (semen-derived enhancer of viral infection) [11] . Mutational and biophysical analysis showed that SEVI, PAP85-120 and SEM fibrils have a positive surface charge that overcomes the electrostatic repulsion between negatively charged virions and cells. This leads to increased rates of viral attachment, fusion and infection [14] , [17] , [20] , [23] . Amyloid-mediated enhancement of HIV infection is highly efficient as in the presence of these fibrils only one to three viral particles are sufficient to establish productive infection in cell culture [11] , [20] . Altogether, these findings suggest that amyloids in semen are essential for the sexual spread of HIV, and that antagonizing their enhancing activity represents an attractive strategy to prevent virus transmission. Several compounds that inhibit assembly of PAP248-286 into SEVI fibrils or prevent the interaction of amyloid with viral particles or cells have been described and are being evaluated for further development as anti-HIV microbicides [12] , [14] , [15] , [16] , [24] , [25] , [26] , [27] . The findings described above come with the caveat that the presence of amyloid fibrils in semen has never been demonstrated. The two amyloidogenic PAP fragments were isolated from a semen-derived peptide library by chromatographic purification of fractions with HIV-enhancing activity [11] , [20] . Amyloid-forming fragments of semenogelins were identified through the use of an antibody recognizing the amyloid fold combined with in silico prediction of protease cleavage [17] . Thus, the presence, structure and functionality of endogenous amyloid in ejaculates remained elusive. Here, we use amyloid-specific dyes and antibodies combined with microscopy-based techniques to demonstrate that amyloid fibrils that bind HIV particles are detectable in human ejaculate. Our findings establish semen as first human body fluid that naturally contains amyloid fibrils in a non-diseased state. These seminal amyloids may play a physiological role in fertility but are apparently exploited by HIV to increase its infectivity and transmission potential. Detection of amyloid in semen Clinically, amyloids that are associated with neurodegenerative disorders such as Alzheimer’s or Parkinson’s disease are diagnosed using amyloid-specific probes that react with the cross β-sheet structure of these fibrils 28,29 . The most commonly applied reagent is Congo red, which makes amyloid appear apple-green under polarized light. Another widely used probe is the benzothiazole salt thioflavin T (ThT), which displays enhanced fluorescence after binding to amyloid. As previously reported 11,30 , high background signals of semen treated with Congo red and ThT prevented the detection of endogenous amyloid by polarization microscopy or fluorescence spectroscopy, respectively. In this study, we therefore sought to apply confocal microscopy that eliminates out-of-focus signals 31 and employed the commercially available amyloid staining kit Proteostat, which contains a 500 nm excitable red fluorescent molecular rotor dye 32 . In total, we analysed ejaculates from 32 healthy donors. For logistical reasons, all samples were allowed to liquefy for 30 min, frozen and stored at −20 °C, defrosted rapidly and incubated with Proteostat. Strikingly, we detected fluorescent amyloid structures in all analysed semen samples ( Fig. 1a,c , Supplementary Fig. 1 ). The number of stained structures varied from 2 to 122 per mm 2 (mean 40±25 per mm 2 ) between donors ( Fig. 1a and Supplementary Fig. 1 ). Endogenous fibrils had a similar size distribution as in vitro grown SEVI fibrils, with the majority of the fibrils being smaller than 100 μm 2 ( Fig. 1b ). 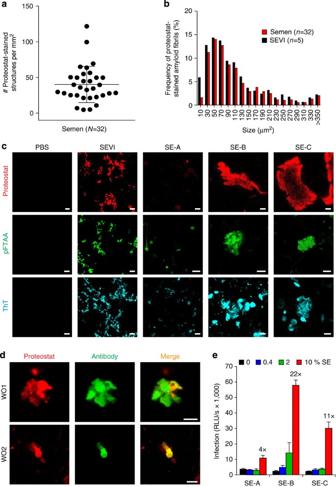Figure 1: Detection of endogenous amyloid in human semen with fluorescent dyes and fibril-specific antibodies. (a) Number of Proteostat-stained structures in semen from individual donors. Liquefied ejaculates were stained with the amyloid-specific Proteostat dye at room temperature for 15–20 min and imaged using a LSM710 confocal microscope. (b) Size distribution of endogenous amyloid in semen, andin vitro-generated SEVI fibrils in buffer. (c) Confocal microscopy images ofin vitro-generated SEVI fibrils and of semen samples (SE-A to SE-C) stained with amyloid-specific probes Proteostat, pFTAA and ThT. Scale bar, 5 μm. PBS, negative control. (d) Detection of amyloid fibrils in semen using amyloid-specific conformational antibodies. Semen was treated with WO1 and WO2 antibodies, and then amyloid/antibody complexes were pelleted, washed and detected using an Alexa488-coupled appropriate secondary antibody (green) and counterstained with Proteostat dye (red). Scale bar, 5 μm. (e) Effect of semen samples A-C on HIV infection. R5-tropic HIV-1 was exposed to indicated concentrations of semen (%) and used to infect TZM-bl cells. After 2 h, semen-virion mixtures were replaced with fresh medium. HIV-1 infection rates were measured 3 days later by quantifying β-galactosidase activities in cell lysates. Values shown are average values derived from triplicate infection±s.d. The numbers above the columns give then-fold enhancement of infection observed after treatment with 10% semen relative to infection with mock-treated virus. Figure 1: Detection of endogenous amyloid in human semen with fluorescent dyes and fibril-specific antibodies. ( a ) Number of Proteostat-stained structures in semen from individual donors. Liquefied ejaculates were stained with the amyloid-specific Proteostat dye at room temperature for 15–20 min and imaged using a LSM710 confocal microscope. ( b ) Size distribution of endogenous amyloid in semen, and in vitro -generated SEVI fibrils in buffer. ( c ) Confocal microscopy images of in vitro -generated SEVI fibrils and of semen samples (SE-A to SE-C) stained with amyloid-specific probes Proteostat, pFTAA and ThT. Scale bar, 5 μm. PBS, negative control. ( d ) Detection of amyloid fibrils in semen using amyloid-specific conformational antibodies. Semen was treated with WO1 and WO2 antibodies, and then amyloid/antibody complexes were pelleted, washed and detected using an Alexa488-coupled appropriate secondary antibody ( green ) and counterstained with Proteostat dye ( red ). Scale bar, 5 μm. ( e ) Effect of semen samples A-C on HIV infection. R5-tropic HIV-1 was exposed to indicated concentrations of semen (%) and used to infect TZM-bl cells. After 2 h, semen-virion mixtures were replaced with fresh medium. HIV-1 infection rates were measured 3 days later by quantifying β-galactosidase activities in cell lysates. Values shown are average values derived from triplicate infection±s.d. The numbers above the columns give the n -fold enhancement of infection observed after treatment with 10% semen relative to infection with mock-treated virus. Full size image To further analyse these seminal amyloids, ejaculates 6 (SE-A), 19 (SE-B) and 27 (SE-C) (see Supplementary Fig. 1 ) were selected because relatively large volumes of these specimens were available and they were representative for ejaculates containing low (SE-A) and normal (SE-B and SE-C) quantities of fibrils ( Fig. 1c ). To confirm the findings obtained with the Proteostat dye, the three ejaculates were incubated with another amyloid-specific probe, the oligothiophene pFTAA [33] . Again, confocal microscopy allowed detection of fluorescent structures resembling those obtained by Proteostat, with relatively small aggregates being present in SE-A, and larger ones in SE-B and SE-C ( Fig. 1c ). Of note, the Proteostat and pFTAA signals co-localized, demonstrating that two chemically divergent amyloid-specific probes recognize similar structures in semen ( Supplementary Fig. 2 ). Finally, confocal microscopy analysis of the three ejaculates treated with ThT provided additional evidence for the presence of endogenous amyloids in these samples ( Fig. 1c ). To verify the findings obtained with the amyloid-specific dyes, we took advantage of the antibodies WO1 and WO2, which recognize a generic amyloid epitope specific for mature amyloid fibrils [34] . Both antibodies readily recognized in vitro -generated SEVI amyloid ( Supplementary Fig. 3 ) and discrete structures in semen that costained with the Proteostat dye ( Fig. 1d ). These results demonstrate that amyloid aggregates are readily detectable in human semen. Finally, we examined the potency of SE-A, -B and -C in enhancing HIV infection. For this, we treated viral particles with the indicated concentrations of semen and then inoculated TZM-bl reporter cells. Determination of infection rates 3 days later revealed that SE-A (containing the lowest quantity of amyloid) enhanced infection less efficiently than SE-B and SE-C ( Fig. 1e ). However, infectivity enhancement did not correlate with the number of Proteostat-stained structures ( Supplementary Fig. 1 ), suggesting both quantitative and functional differences in amyloid fibrils from different donors. Detection of amyloid in fresh semen To clarify whether the freeze/thaw step before semen analysis affects fibril formation, the number of Proteostat and pFTAA-stainable structures in fresh ejaculates and frozen aliquots from the same samples were determined. We detected no significant differences in the number of amyloids in fresh and frozen semen ( Supplementary Fig. 4a,b ). Furthermore, fresh and frozen semen obtained from the same donor promoted HIV infection with similar efficiency ( Supplementary Fig. 4c ). Thus, the freezing procedure has no effect on semen's amyloid content or its viral-enhancing activity. Semen from HIV-infected individuals contains amyloid Thus far, all studies on seminal amyloids have been performed with ejaculates from uninfected donors [11] , [13] , [14] , [15] , [17] . To clarify whether amyloid is also present in semen from infected individuals, we analysed ejaculates obtained from four treatment naive, viremic HIV-1-infected men with at least 5,000 copies per ml HIV-1 RNA in blood plasma and reduced CD4 T-cell numbers. We found that these specimens contained amyloid structures and enhanced HIV-1 infection ( Supplementary Fig. 5 ). High-resolution analysis of endogenous amyloid in semen Amyloid aggregates or deposits consist of individual fibrils that cannot be resolved by confocal microscopy. For direct visualization of fibrils in semen, we subjected SE-A, -B and -C and in vitro grown SEVI fibrils to transmission electron microscopy (TEM). This technique allowed high-resolution imaging of mature amyloid fibrils in SE-B and SE-C, while SE-A contained only low quantities of small amyloid-like structures ( Fig. 2a and Supplementary Fig. 6 ). Amyloid fibrils in SE-B and SE-C often appeared as a dense network of several fibrils arranged side-by-side reaching diameters of more than 15 μm. To examine the structure of seminal fibrils in SE-B and SE-C, their three-dimensional profile was determined by atomic force microscopy (AFM). Images shown in Fig. 2b depict individual fibrils that were between 0.5–2 μm in length and 5–20 nm in diameter, and closely resembled those of in vitro -generated SEVI ( Fig. 2b ). Thus, liquefied human ejaculates contain mature amyloid fibrils. 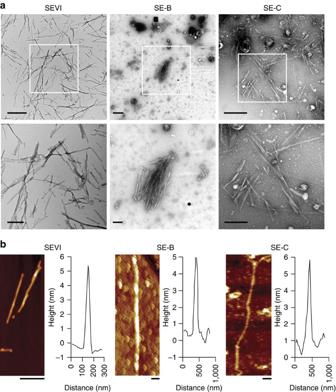Figure 2: Ultrastructural analyses of endogenous amyloid in semen. (a) Transmission electron micrographs of semen.In vitro-generated SEVI fibrils or semen samples SE-B and SE-C were dropped onto EM grids, which were then washed with PBS after 5 min, and then negatively stained with 2% uranyl acetate. All samples were immediately analysed. Scale bars indicate 500 nm for top panel images and 200 nm for bottom panel images. (b) Atomic force micrographs of synthetic SEVI fibrils and endogenous fibrils in semen samples SE-B and SE-C, which were placed on silicon substrates, washed with H2O and imaged in air. Scale bar, 200 nm. The height profiles represent the averages of multiple cross-sections along the fibrils. Figure 2: Ultrastructural analyses of endogenous amyloid in semen. ( a ) Transmission electron micrographs of semen. In vitro -generated SEVI fibrils or semen samples SE-B and SE-C were dropped onto EM grids, which were then washed with PBS after 5 min, and then negatively stained with 2% uranyl acetate. All samples were immediately analysed. Scale bars indicate 500 nm for top panel images and 200 nm for bottom panel images. ( b ) Atomic force micrographs of synthetic SEVI fibrils and endogenous fibrils in semen samples SE-B and SE-C, which were placed on silicon substrates, washed with H 2 O and imaged in air. Scale bar, 200 nm. The height profiles represent the averages of multiple cross-sections along the fibrils. Full size image Endogenous seminal amyloids are in part composed of SEVI We next examined whether endogenous amyloids may be composed of SEVI fibrils. Control experiments showed that an antiserum raised against SEVI [13] , but not the preimmune serum, reacted specifically with in vitro -generated Proteostat-labelled SEVI fibrils ( Supplementary Fig. 7 ). Similarly, the SEVI antiserum recognized structures in semen that costained with the amyloid probe ( Fig. 3a ). Not all of the material that was stained with Proteostat, however, was also recognized by the SEVI antiserum ( Fig. 3a ). Thus, in agreement with previous results [11] , [17] , [20] , our data provide evidence that endogenous amyloids consist of fibrils formed by multiple types of peptides. To verify the fibrillar nature of the structures recognized by the SEVI antiserum, we performed TEM on semen treated with immunogold-labelled SEVI antiserum. As shown in Fig. 3b , gold-conjugated anti-SEVI antibodies specifically bound to fibrils in semen, providing evidence that endogenous SEVI fibrils exist in ejaculates. Thus, endogenous amyloid fibrils consist of PAP248-286 or closely related peptides. 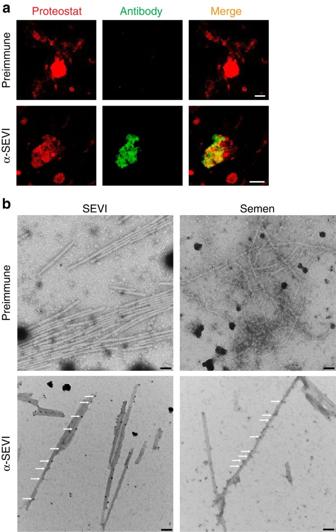Figure 3: Endogenous amyloids partially consists of SEVI. (a) Semen was treated with preimmune (top) or anti-SEVI antiserum (α-SEVI, bottom). The amyloid/antibody complexes were pelleted, washed and incubated with an Alexa488-coupled secondary antibody (green), and counterstained with Proteostat dye (red). Scale bar, 5 μm. (b) Immunogold labelling of endogenous SEVI fibrils in semen. Transmission electron micrographs of semen treated with a preimmune serum or an anti-SEVI antiserum as primary antibodies, and gold-conjugated anti-rabbit secondary antibody. Scale bar, 100 nm. White arrows indicate gold particles bound to amyloid fibrils. Figure 3: Endogenous amyloids partially consists of SEVI. ( a ) Semen was treated with preimmune (top) or anti-SEVI antiserum (α-SEVI, bottom). The amyloid/antibody complexes were pelleted, washed and incubated with an Alexa488-coupled secondary antibody (green), and counterstained with Proteostat dye (red). Scale bar, 5 μm. ( b ) Immunogold labelling of endogenous SEVI fibrils in semen. Transmission electron micrographs of semen treated with a preimmune serum or an anti-SEVI antiserum as primary antibodies, and gold-conjugated anti-rabbit secondary antibody. Scale bar, 100 nm. White arrows indicate gold particles bound to amyloid fibrils. Full size image Endogenous semen amyloids bind HIV particles It has previously been shown that in vitro -assembled PAP and SEM peptides directly interact with HIV particles [11] , [17] , [20] . To study the possible interaction of endogenous seminal amyloid with HIV, Proteostat-stained semen was incubated with EYFP-tagged retroviral particles and analysed by laser scanning confocal microscopy. We observed that seminal amyloid bound all virions within few minutes ( Fig. 4 , Supplementary Movie 1 ). Notably, not all Proteostat-stained structures interacted with virions ( Supplementary Fig. 8 ), and this did not change even under conditions of excess virus ( Supplementary Fig. 9 ), suggesting that HIV may preferentially bind to specific subsets of endogenous amyloid fibrils. It has previously been shown that the polycationic surface charge of synthetic semen fibrils is necessary for virion binding [14] . To test whether similar electrostatic interactions occur between endogenous amyloids and viruses, semen was treated with the polyanion heparin before addition of the virions. As shown in Fig. 4 , the polyanion prevented the formation of amyloid/virus complexes showing that endogenous and synthetic semen amyloids enhance viral infection by a similar mechanism. Finally, pretreatment of HIV-1 virions with fibronectin did not impair the ability of semen to boost HIV infection, demonstrating that this abundant seminal glycoprotein does not prevent the formation of virion/fibril complexes ( Supplementary Fig. 10 ). 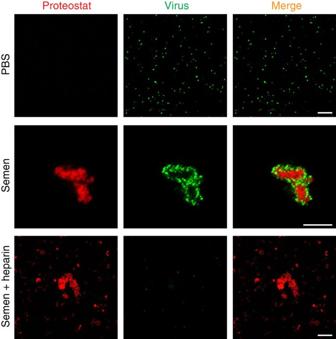Figure 4: Seminal amyloid interacts with retroviral particles. EYFP-labelled virions (green) were mixed with PBS or semen that was stained with Proteostat dye (red). Images were acquired 15 min later on a laser scanning confocal microscope. Single-plane images from the centre of theZ-stack are shown. Treatment of semen with heparin (100 μg ml−1) abrogates the ability of seminal amyloid to bind viral particles. Scale bar, 5 μm. Also seeSupplementary Movie 1. Figure 4: Seminal amyloid interacts with retroviral particles. EYFP-labelled virions (green) were mixed with PBS or semen that was stained with Proteostat dye (red). Images were acquired 15 min later on a laser scanning confocal microscope. Single-plane images from the centre of the Z -stack are shown. Treatment of semen with heparin (100 μg ml −1 ) abrogates the ability of seminal amyloid to bind viral particles. Scale bar, 5 μm. Also see Supplementary Movie 1 . Full size image In this study, we provide multiple lines of evidence for the presence of amyloid fibrils in semen. First, liquefied ejaculates obtained from healthy donors contained aggregates that stained with three different amyloid-specific fluorescent probes ( Fig. 1c ). Second, the two unrelated amyloid dyes pFTAA and Proteostat bound to the same structures ( Supplementary Fig. 2 ) thus precluding unspecific staining of non-amyloid semen components. Third, amyloid-specific antibodies, which have previously been used to detect amyloid in vivo, specifically recognized aggregates in semen that costained with Proteostat ( Fig. 1d ). Finally, typical amyloid fibrils were directly detected in ejaculates by TEM and AFM analyses ( Figs 2 and 3 ). These findings establish semen as body fluid that naturally contains amyloid. In striking contrast to the well-known insoluble amyloid deposits associated with severe disorders like Alzheimer’s disease, seminal amyloids exist in dispersion and are present in ejaculates derived from healthy individuals. Their physiological relevance remains to be determined, but it is tempting to speculate that they may play a role in reproduction. In either case, our results substantially change the present view about amyloids as harmful debris. Using confocal microscopy analysis of pure semen, we found that endogenous amyloids bind viral particles resulting in a local enrichment of the virions at the amyloid surface ( Fig. 4 , Supplementary Movie 1 ). Virus-loaded fibrils can then bind to the cell surface and efficiently establish infection [11] , [14] , [15] , [17] , [20] , [23] . The formation of amyloid/virus complexes occurs rapidly (within seconds to minutes) and is highly efficient as most if not all virions are trapped by amyloid. This provides an explanation for why only one to three infectious particles are sufficient to establish a productive infection in the presence of SEVI or PAP85-120 fibrils, in comparison with the thousands of virions required in the absence of fibrils [11] , [20] . The unambiguous detection of HIV-binding amyloid in semen from uninfected and HIV-infected individuals further supports its previously proposed role in the sexual spread of the AIDS pandemic [11] , [12] , [13] , [14] , [15] , [16] , [17] , [18] , [19] , [20] . If the HIV-enhancing effect of semen amyloids applies to the in vivo situation, antagonizing this activity may represent a novel strategy to prevent sexual transmission of HIV and eventually other enveloped viruses such as cytomegalovirus [35] . Several inhibitors of SEVI and semen-mediated enhancement of HIV infection have been described and are currently evaluated as candidates for microbicide development [12] , [14] , [15] , [16] , [24] , [25] , [26] , [27] . However, it is important to consider that compounds that antagonize the HIV-enhancing activity of amyloid in semen might also interfere with its normal physiological function. Current amyloid detection protocols have been developed to diagnose amyloid deposits in biopsied tissues or to study purified or synthetic fibrils in buffered solutions [28] , [29] . We have previously applied Congo red staining of semen but did not observe amyloid-specific green birefringence by polarization microscopy, the most recognized diagnostic procedure to detect amyloid in vivo . Although the reasons for this are currently unclear, it seems likely that Congo red either does not bind to dispersed seminal amyloid, or that seminal amyloid stained with this reagent does not cause green birefringence, as it has been reported before for functional amyloid in melanosomes [36] . A second routinely used technique to determine and quantify amyloid is fluorescence spectroscopy, which measures changes in the fluorescence intensity of ThT upon binding to amyloid fibrils [28] , [29] . However, high background levels caused by unspecific binding of ThT to semen components prevented utilization of this methodology for detection of semen amyloids [11] , [30] . To overcome these caveats, we applied laser scanning confocal microscopy, which collects fluorescence only from the focal plane leading to reduced background signals and enhanced spatial resolution. This approach allowed us to detect fluorescent structures after staining with different amyloid-specific probes. The number, morphology and size of amyloids varied substantially between individual semen samples. For instance, some ejaculates contained high numbers (~120 per mm 2 ) of relatively small amyloid aggregates (~30 μm 2 ), while others contained lower numbers (~5 per mm 2 ) of larger size fibrils (>300 μm 2 ). Interestingly, however, the average size distribution of amyloid in semen was very similar to that obtained for synthetic SEVI fibrils ( Fig. 1b ). Thus, endogenous and synthetic fibrils have similar length and width distributions. The exact composition and concentrations of semen amyloid remain to be determined, but they are at least in part made up of PAP248-286 or closely related peptides. Of note, semen apparently also contains amyloid fibrils that do not sequester viral particles ( Supplementary Fig. 8 ), suggesting the presence of other amyloid species. The normal physiological role of amyloids in semen remains unknown. It has recently been reported that synthetic SEVI fibrils have an indirect antimicrobial activity because they form a positively charged ‘mesh’ that is capable of trapping microbial pathogens [37] . Subsequently, the aggregated bacterial/fibril complexes are phagocytosed by primary macrophages and thus cleared. However, evidence that endogenous amyloids are also part of the innate immune defence is missing. Given that semen’s main purpose is to protect and provide nutrients for spermatozoa, it is tempting to speculate that seminal amyloids are involved in sperm cell function and/or fertilization. Future studies aiming at elucidating the natural role of semen amyloids are thus highly warranted and may provide new insights in human reproduction. Human semen samples De-identified semen samples from HIV-seronegative individuals were obtained, following informed consent, from adult donors presenting at the ‘Kinderwunsch-Zentrum Ulm’, a fertility centre in Ulm, Germany. After ejaculation, samples were allowed to liquefy for approximately 30 min, pipetted and frozen at −20 °C. Liquefaction is a normal property of semen that takes place after ejaculation and results in the release of spermatozoa. All experiments were performed with freshly thawed aliquots and were approved by the local ethics committee at Ulm university (proposal numbers 351/10 and 156/13). Semen from HIV-1-infected individuals was donated following informed consent by participants in the UCSF Options study, a cohort of HIV-infected men in San Francisco, USA. At the time of donation, median (and range) values for CD4 cell count and HIV viral load were 390 (150–980) CD4 cells mm −3 and 4.5 (3.7–5.1) log10 HIV-1 RNA copies per ml of blood plasma, respectively. No subjects were on antiretroviral therapy at the time of specimen donation. This study was approved by UCSF Human Research Protection Program, study number 10-00301. Peptides and amyloid formation PAP248-286 peptide was obtained from Celtek Peptides (Nashville, USA). Amyloid formation was induced by agitating 10 mg ml −1 solutions in PBS in an Eppendorf Thermomixer over night at 37 °C at 1,400 r.p.m. Cell culture HEK293T cells were obtained from ATCC (CRL-11268), and TZM-bl indicator cells were obtained from the NIH AIDS Reagent Program (Catalogue Number 8129). Cells were grown in DMEM containing 10% FCS and antibiotics. Detection of amyloid in semen using the ProteoStat detection kit The ProteoStat Amyloid Plaque Detection Kit (ENZ-51038-K040, Enzo Life Science, Germany) was used as recommended by the manufacturer. Fresh and frozen/thawed ejaculates were stained with Proteostat dye at room temperature for 15–20 min. Semen from HIV-1-infected men were first treated with 2% paraformaldehyde for 30 min before staining. Stained semen was then transferred onto μ-Slide VI Ibidi slides (IbidiGmbH). As a positive control, 100 μg ml −1 SEVI was simultaneously stained and analysed. The dye was excited by using a 561 nm laser line, and the emission was collected using appropriate beam splitters. For acquiring images, Plan-Apochromat × 63/1.40 oil objective lenses on a LSM710 confocal microscope (Zeiss) equipped with Zen-Software (Zeiss, Germany) was used. The confocal pin hole was adjusted to 1 airy unit. For counting fluorescent aggregates in semen, at least 5 images were acquired from different regions for every stained sample. Images were processed using the Zen-Software (Zeiss, Germany). Quantification of Proteostat-stained structures in semen To quantify microscopy data obtained from Proteostat-stained semen samples, at least five images were analysed from each sample. Before performing analysis, background fluorescence was subtracted from the images. To further exclude non-specific staining and stained spermatozoa and cells, only stained structures that were larger than 2 × 2 μm were enumerated using FIJI software. To measure the area, mean intensity and integrated density of Proteostat-stained structures, a region of interest was drawn around fluorescent structures and calculation was performed in FIJI. Frequency distribution was performed using GraphPad Prism. Similar analysis was performed with 100 μg ml −1 Proteostat-stained SEVI fibrils. Detection of amyloid in semen using Thioflavin T and pFTAA Semen samples were incubated with 10 μM ThT or 1 μM luminescent-conjugated oligothiophene dye pFTAA for 15–30 min. ThT was excited by using a 405 nm laser line, and the emission was collected using an MBS-405 beam splitter. pFTAA was excited by using a 488 nm laser line, and the corresponding emission was collected using an MBS-488 beam splitter. Confocal images were acquired using Plan-Apochromat × 63/1.40 oil objective lenses on a LSM710 confocal microscope (Zeiss) equipped with Zen-Software 2010 (Zeiss, Germany). The confocal pin hole was adjusted to 1 airy unit. Images were processed using the Zen-Software 2010 (Zeiss, Germany). Detection of seminal amyloid with amyloid-specific antibodies Liquefied ejaculates (100 μl) were mixed with 0.5% fish skin gelatin containing PBS. To this mixture, 100 nM WO1 or WO2 antibodies, or 500-fold dilution of a preimmune serum or an anti-SEVI antiserum was added and incubated for 3–4 h at 4 °C. The antibody–amyloid complexes were pelleted at 13,000 r.p.m. for 10 min, washed twice with PBS and pelleted again. The pellet was then dissolved in 0.5% fish skin gelatin containing PBS and treated with an Alexa488 conjugated secondary antibody for 3 h. The mixture was pelleted again, dissolved in PBS and counterstained with Proteostat. Confocal images were acquired as described above. Transmission electron microscopy of individual semen samples Five microlitres of semen was dropped onto the EM copper grid. After 5 min, excess semen was removed with a Whatmann filter paper, followed by a PBS wash step. The grid was stained with 2% uranyl acetate for 2 min, and remaining uranyl acetate was removed with Whatmann filter paper. The grid was washed three times with water and then air dried. Samples were imaged with a Zeiss EM 10 transmission electron microscope at an accelerating voltage of 80 kV. Immunogold labelling for transmission electron microscopy Five microlitre droplets of semen or preformed SEVI fibrils were placed on a Formvar-coated copper grid (Ted Pella Inc.) and incubated for 5 min. The grid was washed three times (10 s each) with 50 μl droplets of PBS, pH 7.4 (1 × Dulbecco’s PBS, Sigma Aldrich). Excess solvent was carefully soaked off with filter paper before a 50 μl droplet of 5% bovine serum albumin in PBS was applied for 15 min. Afterwards the grid was washed with a droplet of 50 μl buffer. Excess solvent was removed with filter paper, and the grid was incubated for 1 h with either 50 μl of anti-SEVI antiserum or respective preimmune serum (both diluted 1:100 in PBS) and covered by a Petri dish. The grid was washed in PBS as described above, before a 50 μl droplet of goat anti-rabbit antibody conjugated to 10 nm gold particles (Sigma Aldrich, 1:100 dilution in PBS) was applied. The grid was then washed again with a 50 μl droplet of PBS containing 0.05% Tween 20 for 20 s and three droplets of 50 μl water for 10 s each. Finally, the grid was stained using a series of three 50 μl droplets containing 2% uranyl acetate (20 s each) and then dried with filter paper. All steps were carried out at room temperature. Semen samples labelled with an anti-SEVI antiserum and respective preimmune serum were examined under a Zeiss 900 electron microscope, operated at an acceleration voltage of 80 kV. Atomic force microscopy analysis An aliquot of 5 μl of freshly thawed semen or preformed SEVI fibrils was placed on a freshly cleaned (isopropanol, H 2 O) Silicon surface. After incubation for 5 min, the substrates were rinsed with 1 ml H 2 O and dried in air. Samples were measured under ambient conditions using a Nanoscope IIIa (Digital Instruments) utilizing silicon cantilevers with a spring constant of 2 N/m (Olympus). The images were analysed using SPIP 5 software (Image Metrology). Interaction of endogenous amyloids with virions EYFP-Gag virions were produced by transfection of 293T cells with MLV Gag-EYFP and MLV-Gag-Pol expression plasmids at a 1:10 ratio using the calcium chloride method [11] . Two days after transfection, supernatants were collected and virions were concentrated by ultracentrifugation at 15,000 g for 2 h at 4 °C. Semen was stained with Proteostat and incubated with EYFP- tagged virions for 15 min at RT. Z -stack images were acquired with a LSM710 confocal microscope (Zeiss). Proteostat dye fluorescence was assessed as described above, while EYFP was excited by using a 514 nm laser line, and the corresponding emission was collected using an MBS 458/514 beam splitters, using Plan-Apochromat × 63/1.40 Oil objective lens. Effect of semen on HIV-1 infection A total of 1 × 10 4 TZM-bl cells were seeded in microtitre plates in a volume of 280 μl medium (DMEM supplemented with 10% FCS, 100 units per ml penicillin, 100 μg ml −1 streptomycin and 50 μg ml −1 gentamicin). The following day, frozen semen samples were thawed, briefly vortexed and serially diluted fivefold in PBS. Then, 40 μl of these dilutions were transferred to U-bottom microtitre plates and mixed with 40 μl of R5-tropic HIV-1 11 containing 0.1 ng ml −1 p24 antigen. The concentrations of semen during virion treatment were 10, 2, 0.4 and 0%. After 5 min incubation at RT, the HIV/semen mixtures were resuspended and 20 μl were used to infect 280 μl TZM-bl cells. The HIV/semen inoculum was removed after 2 h of incubation, and cells were further cultivated in 200 μl fresh DMEM (supplemented with 10% FCS and antibiotics). Infection rates were measured 3 days later by quantifying β-galactosidase activities using the Gal-Screen assay kit (Applied Biosystem, T1027) according to the manufactureŕs instructions. Luminescence was recorded with an Orion microplate luminometer. How to cite this article: Usmani, S. M. et al. Direct visualization of HIV-enhancing endogenous amyloid fibrils in human semen. Nat. Commun. 5:3508 doi: 10.1038/ncomms4508 (2014).